Srs2 prevents Rad51 filament formation by repetitive motion on DNA Srs2 dismantles presynaptic Rad51 filaments and prevents its re-formation as an anti-recombinase. However, the molecular mechanism by which Srs2 accomplishes these tasks remains unclear. Here we report a single-molecule fluorescence study of the dynamics of Rad51 filament formation and its disruption by Srs2. Rad51 forms filaments on single-stranded DNA by sequential binding of primarily monomers and dimers in a 5′–3′ direction. One Rad51 molecule binds to three nucleotides, and six monomers are required to achieve a stable nucleation cluster. Srs2 exhibits ATP-dependent repetitive motion on single-stranded DNA and this activity prevents re-formation of the Rad51 filament. The same activity of Srs2 cannot prevent RecA filament formation, indicating its specificity for Rad51. Srs2’s DNA-unwinding activity is greatly suppressed when Rad51 filaments form on duplex DNA. Taken together, our results reveal an exquisite and highly specific mechanism by which Srs2 regulates the Rad51 filament formation. DNA in the living cell is subject to many chemical alterations. In human cells, both normal metabolic activities and external insults such as ultraviolet exposure and environmental chemicals can cause DNA damage of various types. DNA double-strand breaks are the principal cytotoxic damage repaired by homologous recombination (HR), which is mediated by the Rad51 recombinase in eukaryotes [1] , [2] . However, unrepaired double-strand breaks give rise to harmful mutations and chromosome rearrangements that lead to carcinogenesis. Mutations found in BRCA1 and BRCA2 (breast cancer susceptibility gene 1 and 2), which have a critical role in DNA repair, confer an elevated risk for breast and ovarian cancer, underscoring the significance of DNA repair in tumour suppression. Therefore, specific mechanisms have evolved to regulate HR and to minimize deleterious outcomes [3] , [4] , [5] . In the budding yeast Saccharomyces cerevisiae , Srs2 is one of the major HR regulators that functions in the early stages of the HR pathway. Srs2 is an ATP-dependent 3′–5′ DNA helicase and single-stranded DNA (ssDNA) translocase [6] that prevents HR by dismantling Rad51 filaments [7] , [8] , [9] . Such anti-recombinase activity is crucial for preventing accumulation of genotoxic intermediates and chromosomal aberration [10] . Srs2 mutants that cannot bind or hydrolyse ATP fail to disrupt Rad51 filaments and display a hyper-recombination phenotype when subjected to genotoxic stress [11] . This anti-recombinase activity requires direct interaction of Srs2 with Rad51 and may require Srs2 translocation along ssDNA [6] . Consistent with this view, Srs2 cannot remove a Rad51 mutant that lacks the Srs2 interaction domain [12] , [13] . The same mechanism may be preserved in the human helicase RECQ5, which also disrupts human Rad51 (hRad51) filaments via direct physical contact [10] . In this study, we used single-molecule fluorescence to investigate the molecular mechanism controlling the balance between Rad51 filament formation and disruption by Srs2. Using single-molecule Förster resonance energy transfer (FRET), we find the Rad51 site size to be three nucleotides and its nucleation size to be six monomers. We employed an alternative detection method, protein-induced fluorescence enhancement (PIFE) [14] , [15] , [16] to determine the Rad51 loading directionally from 5′ to the 3′. We also report a novel repetitive motion of Srs2 monomer that prevents re-formation of Rad51 filaments. This activity occurs after the initial clearance of Rad51, hence contributes to the anti-recombinase function of Srs2. Finally, the DNA-unwinding activity of Srs2, which requires multimers of Srs2, was greatly diminished by Rad51 bound to duplex DNA, indicating a further balance between the helicase and anti-recombinase activity of Srs2. Our study reveals novel mechanistic details that govern the early stages of the HR DNA repair pathway. Rad51 has a three-nucleotide-site size To visualize Rad51 filament formation, we prepared DNA substrates that mimic a resected DNA intermediate found during HR, which is the preferred substrates for Rad51 formation and strand invasion [17] . They are partial DNA duplexes with variable lengths of 3′-ssDNA composed of poly deoxythymidine, T10, 13, 15, 18 and 20, referred to as pdT10–pdT20 hereafter ( Fig. 1a ). Each DNA possesses two fluorophores, Cy3 and Cy5, located at the 3'-end of the ssDNA and at the duplex DNA end, respectively ( Fig. 1a ), such that DNA alone exhibits high FRET owing to the high flexibility of the ssDNA [18] and low FRET upon Rad51 binding. The histograms of FRET values built from over 5,000 molecules of DNA show FRET peaks at around 0.85, 0.8, 0.75, 0.7 and 0.65 for pdT10, 13, 15, 18 and 20, respectively ( Fig. 1b , grey). Upon addition of Rad51 (1 μM) and ATP (1 mM), the high FRET peaks disappear and another low FRET population arises, indicating formation of Rad51 filaments on ssDNA ( Fig. 1b , orange histograms). The complete shift from high to low FRET observed for pdT18 and pdT20 indicates formation of stable Rad51 filaments, whereas the partial shift seen for pdT15 and shorter ssDNA suggests a less stable filament. 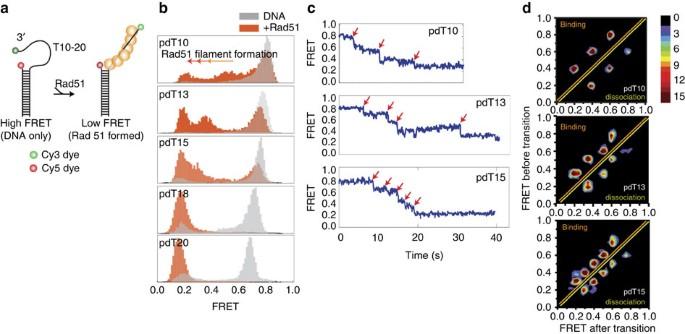Figure 1: Rad51 monomer binds three nucleotides and stable nucleation requires six monomers. (a) Schematic diagram of DNA constructs used in Rad51-binding experiment. Partially duplexed DNA of various poly-thymidine tail lengths (T10–T20) contain donor (Cy3) at 3′-end and acceptor (Cy5) at duplex junction. FRET value decreases upon Rad51 formation. (b) FRET values collected over 5,000 single molecules are built into a FRET histogram. DNA-only high FRET molecules (grey) transition to low FRET (orange) upon Rad51 formation. A complete shift to low FRET is observed in T18 and T20. (c) smFRET traces show up to three, four and five steps observed for T10, T13 and T15, respectively, reflecting monomer-binding steps. (d) TDP for each DNA built by collecting FRET values before (yaxis) and after (xaxis) transition from single molecules that show monomer-binding steps. Figure 1: Rad51 monomer binds three nucleotides and stable nucleation requires six monomers. ( a ) Schematic diagram of DNA constructs used in Rad51-binding experiment. Partially duplexed DNA of various poly-thymidine tail lengths (T10–T20) contain donor (Cy3) at 3′-end and acceptor (Cy5) at duplex junction. FRET value decreases upon Rad51 formation. ( b ) FRET values collected over 5,000 single molecules are built into a FRET histogram. DNA-only high FRET molecules (grey) transition to low FRET (orange) upon Rad51 formation. A complete shift to low FRET is observed in T18 and T20. ( c ) smFRET traces show up to three, four and five steps observed for T10, T13 and T15, respectively, reflecting monomer-binding steps. ( d ) TDP for each DNA built by collecting FRET values before ( y axis) and after ( x axis) transition from single molecules that show monomer-binding steps. Full size image Representative single-molecule FRET (smFRET) traces show a stepwise FRET decrease, possibly representing the sequential binding of Rad51 molecules ( Fig. 1c ). For pdT10, 13 and 15, a maximum of three, four and five steps of FRET decrease were observed, suggesting the binding of up to three, four and five Rad51 monomers. We collected FRET values from 40 to 50 single-molecule traces that display clear steps and built a transition density plot (TDP) where the y and x axes represent FRET before and after the transition, respectively. Here, three, four and five peaks are observed in the TDP for T10, 13 and 15, respectively, above the diagonal line ( Fig. 1d ), reflecting one Rad51 monomer binding to three nucleotides, consistent with the crystal structure of the Rad51 [19] and RecA–ssDNA filament [20] , [21] . Because of the unstable binding of Rad51 to these shorter lengths of ssDNA, we obtained mirror image peaks below the diagonal line, reflecting dissociation of Rad51. This set of data suggests that a Rad51 monomer binds three nucleotides of ssDNA and that six monomers are required to form a stable nucleation cluster. In addition to the monomer binding, we also observe larger steps of FRET decrease and increase, representing binding and dissociation, respectively, of larger Rad51 oligomers ( Supplementary Fig. S1b ). On the basis of the well-defined FRET states mapped for monomer Rad51, the observed FRET values were assigned as monomers to tetramers ( Supplementary Fig. S1a–c ). The analysis suggests that ~75% of Rad51 binds as either a monomer or dimer to pdT15 ( Supplementary Fig. S1d ). Rad51 filaments form in the 5′–3′ direction Next, we examined the directionality of Rad51 filament formation. Ensemble stopped-flow experiments suggest a 5′–3′ directional bias for Rad51 filament formation on ssDNA without a duplex junction [6] . We tested it on resected DNA intermediate. Although FRET is useful for visualizing monomer binding, it does not inform us about the directionality (for example, growing from 3′ to 5′ or 5′ to 3′). We took advantage of an alternative fluorescence method, single-molecule PIFE (smPIFE) whereby the intensity of a Cy3 fluorophore increases upon protein binding in its vicinity in a distance-dependent manner [6] , [14] , [15] , [16] . We used two identical DNAs with Cy3 fluorophore located at either the 3′- or near the 5′-end of the ssDNA ( Fig. 2a ). When Rad51 was added, the 3′-labelled DNA showed a multi-step increase ( Fig. 2b ), whereas 5′-labelled DNA showed a single-step increase in Cy3 fluorescence ( Fig. 2c,d ), indicating 5′–3′ extension bias of Rad51 filament. We note that the intensity increase is greater for Cy3 at the 3'-end because the dye is located at a conformationally more flexible position, which is more sensitive to the PIFE effect [22] , [23] . The same pattern is also observed when the intensities of single-molecule traces are averaged and normalized by its minimum ( Fig. 2e ). The 3.3-fold higher rate for the 5′-Cy3 than that compared with the 3′-Cy3 indicates the nucleation initiating preferentially from the 5′-end (duplex junction). Both sets of data are consistent with the initiation of the Rad51 nucleation at the duplex junction and assembly/extension towards the 3′-end of the ssDNA ( Fig. 2f ). Rad51 can also form a filament on double-stranded (ds) DNA [24] , [25] , [26] , but the rate of filament assembly on dsDNA is sixfold lower (0.05 s −1 ) than the rate observed for assembly on ssDNA (0.28 s −1 ; Supplementary Fig. S2a–e ). On the basis of these results, Rad51 binding to dsDNA does not influence the directionality of its nucleation on the ssDNA substrates tested here. 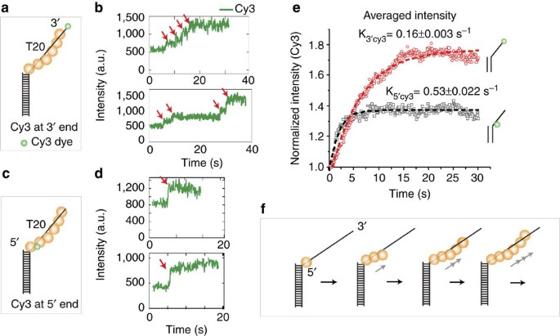Figure 2: Rad51 binds in 5′–3′ direction. (a) Schematic of 3′ Cy3-labelled DNA used in PIFE assay. (b) Single-molecule trace displaying a gradual and stepwise increase in Cy3 signal. (c) Schematic of 5′-Cy3-labelled DNA used in PIFE assay. (d) Single-molecule trace showing an abrupt increase in Cy3 signal. (e) Normalized average intensity plots for both DNA constructs showing slower increase in 3′-Cy3 DNA compared with 5′-Cy3 DNA. Errors in fit results are in s.e.m. (f) Schematic summary of Rad51 binding in 5′–3′ direction. Figure 2: Rad51 binds in 5′–3′ direction. ( a ) Schematic of 3′ Cy3-labelled DNA used in PIFE assay. ( b ) Single-molecule trace displaying a gradual and stepwise increase in Cy3 signal. ( c ) Schematic of 5′-Cy3-labelled DNA used in PIFE assay. ( d ) Single-molecule trace showing an abrupt increase in Cy3 signal. ( e ) Normalized average intensity plots for both DNA constructs showing slower increase in 3′-Cy3 DNA compared with 5′-Cy3 DNA. Errors in fit results are in s.e.m. ( f ) Schematic summary of Rad51 binding in 5′–3′ direction. Full size image Srs2 monomer displays repetitive movement on DNA To probe the translocation activity of Srs2, which is thought to contribute to its anti-recombinase function [6] , we examined its ATP-stimulated movement on pdT20 ( Fig. 3a ). We used a well-characterized C-terminal deletion mutant, Srs2 CΔ276 in all experiments unless stated otherwise. This mutant protein exhibits ATP-driven translocation and anti-recombinase activity [6] , and we refer it as Srs2 from here on. When Srs2 was added with ATP, we obtained single-molecule traces of highly repetitive FRET fluctuations reflecting repeated motion of Srs2 on ssDNA, which induces repetitive distance changes between the two ends of the ssDNA ( Fig. 3b ). These fluctuations require ATP hydrolysis as they are not seen in the absence of ATP or presence of ATPγS ( Supplementary Fig. S3a ). Furthermore, the periodicity measured by collecting dwell times (δ t ) from over 300 events shows a dependence on ATP concentration ( Supplementary Fig. S3b,c ). A fit of these data to the Michaelis–Menten equation yields K m =9.26±1.72 μM ATP and V max =0.64±0.02 s −1 ( Fig. 3c ). To test whether the FRET fluctuations arise from a monomer Srs2 or successive binding of multiple monomers, we tethered a histidine-tagged Srs2 (0.5–1 nM) to a surface treated with biotinylated Ni–NTA (nitroloacetic acid); ( Fig. 3d ) and added Cy3–Cy5-labelled DNA substrate (non-biotinylated). Here we monitored FRET fluctuations, representing the repetitive motion of a Srs2 monomer on ssDNA ( Fig. 3e,f ). The DNA binding is highly specific to the presence of surface-tethered Srs2 as we do not see any fluorescence spots in the absence of Ni–NTA or Srs2. This assay enables us to clearly distinguish the moment of DNA binding as an abrupt appearance of FRET, duration of repetitive motion as a continuous FRET fluctuation (grey bars) and the DNA dissociation as the disappearance of FRET ( Fig. 3e,f ). This provides direct evidence that a monomer of Srs2 is sufficient for the repetitive motion. We note that this activity is not the initial directional translocation of Srs2 on ssDNA, which occurs at a rate of 300 nucleotides per second [6] , which is beyond our time resolution of 30–100 ms, but what occurs after the fast translocation. 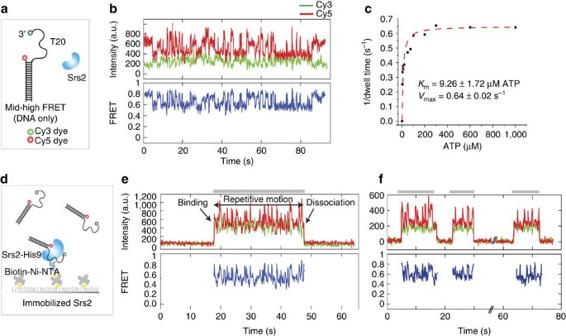Figure 3: Srs2 exhibits repetitive motion on ssDNA. (a) Schematic diagram of FRET–DNA used in Srs2 assay. (b) Single-molecule traces displaying Srs2-induced FRET fluctuation. (c) The inverse of FRET peak-to-peak dwell time was fitted to Michaelis–Menten equation. Errors in fit results are in s.e.m. (d) Schematic diagram of tethered protein assay. Histidine (9 × )-tagged Srs2 was immobilized to surface and non-biotinylated FRET–DNA substrate was applied. (e) Single-molecule traces show that the repetitive motion arises from a single monomer of Srs2. DNA binding, Srs2-mediated repetitive motion and dissociation from Srs2 are shown as an appearance of FRET, FRET fluctuation and disappearance of FRET, respectively. (f) Single-molecule trace shows multiple bursts of repetitive events arising from single Srs2 monomer. Figure 3: Srs2 exhibits repetitive motion on ssDNA. ( a ) Schematic diagram of FRET–DNA used in Srs2 assay. ( b ) Single-molecule traces displaying Srs2-induced FRET fluctuation. ( c ) The inverse of FRET peak-to-peak dwell time was fitted to Michaelis–Menten equation. Errors in fit results are in s.e.m. ( d ) Schematic diagram of tethered protein assay. Histidine (9 × )-tagged Srs2 was immobilized to surface and non-biotinylated FRET–DNA substrate was applied. ( e ) Single-molecule traces show that the repetitive motion arises from a single monomer of Srs2. DNA binding, Srs2-mediated repetitive motion and dissociation from Srs2 are shown as an appearance of FRET, FRET fluctuation and disappearance of FRET, respectively. ( f ) Single-molecule trace shows multiple bursts of repetitive events arising from single Srs2 monomer. Full size image Srs2 displays repetitive motion on ssDNA at ss–ds junction To probe the mechanistic basis of this repetitive action, we varied the lengths of the ssDNA from pdT13 to pdT70 ( Fig. 4a ). We observe similar FRET fluctuations when the tail length is between 13 and 20, with similar amplitude changes as depicted both in single-molecule traces ( Fig. 4b ) and FRET histograms taken from over 100 events ( Fig. 4c ). For 25 and 30 nucleotides, FRET fluctuations occur at a lower FRET range with less pronounced FRET peaks. Such FRET patterns completely disappear for the pdT70 DNA ( Fig. 4b,c ). Dwell time analyses suggest that the fluctuations are not length dependent beyond 20 nucleotides, indicating that the repetitive movement is limited to ~18–20 nucleotides of ssDNA length ( Fig. 4d,e ). Both FRET pattern and dwell time analysis point to a mechanism whereby Srs2, while bound at the junction, periodically reels in a finite segment of ssDNA of ~18–20 nucleotides, rather than the entire length of ssDNA. To test this hypothesis further, we prepared three substrates with tail lengths of pdT30, pdT40 and pdT50, but with each containing two dyes separated by 15 nucleotides ( Supplementary Fig. S4a ). We observe the same FRET fluctuation with similar periodicity for all three DNA substrates ( Supplementary Fig. S4b–d ), consistent with the mechanism described above. Experiments with fluorescently labelled Srs2 further support this model of junction-anchored Srs2 repetitively pulling in the 3′-tail ( Supplementary Fig. S4e–l ). It is interesting to note that this activity involves an apparent 5′–3′-directed movement, opposite of its 3′–5′ directional translocation [6] . 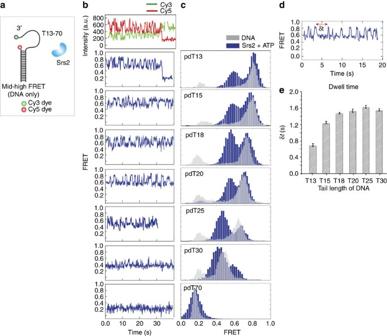Figure 4: Srs2 displays repetitive motion on short segments of ssDNA. (a) Schematic of FRET–DNA constructs with various tail lengths (T13–T70). (b) Single-molecule traces show similar range of FRET fluctuation in T13–T20, but much less prominent and lower FRET range fluctuation in T25–T30 and no fluctuation in T70. (c) FRET histograms of single-molecule traces of Srs2 on various ssDNA tail lengths. (d) FRET peak-to-peak dwell time δt. (e) Dwell times collected from various tail lengths. Error bars denote s.e.m. based on 500 molecules obtained from three independent measurements. Figure 4: Srs2 displays repetitive motion on short segments of ssDNA. ( a ) Schematic of FRET–DNA constructs with various tail lengths (T13–T70). ( b ) Single-molecule traces show similar range of FRET fluctuation in T13–T20, but much less prominent and lower FRET range fluctuation in T25–T30 and no fluctuation in T70. ( c ) FRET histograms of single-molecule traces of Srs2 on various ssDNA tail lengths. ( d ) FRET peak-to-peak dwell time δ t . ( e ) Dwell times collected from various tail lengths. Error bars denote s.e.m. based on 500 molecules obtained from three independent measurements. Full size image Srs2 anti-recombinase activity Next, we tested whether the repetitive activity of Srs2 contributes to its anti-recombinase activity. We formed a Rad51 filament on Cy3–Cy5-labelled pdT20 DNA ( Fig. 5a ) and added Srs2 (20–200 nM) together with Rad51 to maintain the same Rad51 concentration. The representative single-molecule trace shows a steady low FRET transitioning to a high FRET followed by FRET fluctuations, suggesting a complete clearance of the Rad51 filament ( Fig. 5b ). The initial FRET increase corresponds to the dismantling of Rad51 by Srs2 translocation [6] , whereas the FRET fluctuation reflects the repetitive motion of Srs2 that occurs after the removal process. This result suggests that after Srs2 removes Rad51 filament, it stays on the DNA and prevents re-binding of Rad51 by repeatedly pulling in the ssDNA. This can also be advantageous for subsequent binding of replication protein A (RPA) to reinforce the clearance of the Rad51 filament. 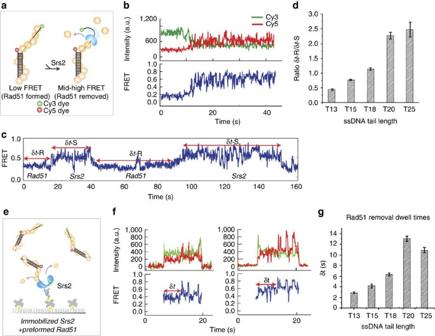Figure 5: Srs2 repetitive motion prevents Rad51 formation. (a) Schematic of FRET–DNA used in Rad51 removal assay. (b) Single-molecule traces showing low-to-high FRET followed by FRET fluctuation. (c) Single-molecule traces displaying dynamic exchange between Rad51 filament formation and Srs2 clearance. (d) Ratio between filament-formed duration and Srs2-cleared duration tested on varying tail. Error bars denote s.e.m. based on 100 events from 40 molecules. (e) Schematic of immobilized Srs2 assay to test whether clearance and repetitive activity arises from Srs2 monomer. (f) Single-molecule traces showing monomer Srs2 removing Rad51 filament and preventing re-formation. (g) Dwell times corresponding to removal duration for different tail length. Error bars denote s.e.m. Figure 5: Srs2 repetitive motion prevents Rad51 formation. ( a ) Schematic of FRET–DNA used in Rad51 removal assay. ( b ) Single-molecule traces showing low-to-high FRET followed by FRET fluctuation. ( c ) Single-molecule traces displaying dynamic exchange between Rad51 filament formation and Srs2 clearance. ( d ) Ratio between filament-formed duration and Srs2-cleared duration tested on varying tail. Error bars denote s.e.m. based on 100 events from 40 molecules. ( e ) Schematic of immobilized Srs2 assay to test whether clearance and repetitive activity arises from Srs2 monomer. ( f ) Single-molecule traces showing monomer Srs2 removing Rad51 filament and preventing re-formation. ( g ) Dwell times corresponding to removal duration for different tail length. Error bars denote s.e.m. Full size image Although the repetitive motion by Srs2 serves to maintain the ssDNA clear of Rad51, this activity is transient, because >60% of single-molecule traces display a dynamic exchange between the steady low FRET and the FRET fluctuations, representing re-formation of Rad51 filaments and subsequent clearance by Srs2, respectively ( Fig. 5c ). To test whether the stability of the Rad51 filament influences its clearance by Srs2, we measured the dwell times corresponding to the duration corresponding to the Rad51-formed state (δ t -R, low FRET) and Srs2-induced clearance (δ t -S, FRET fluctuation; Fig. 5c ) for varying lengths of the ssDNA tail. The ratio between δ t -R and δ t -S, which provides a measure of the propensity for Rad51 filament formation over clearance ( Fig. 5d ), shows that the longest ssDNA (T25) is five times more likely to be occupied by a Rad51 filament than the shortest ssDNA (T13). In other words, the T13 ssDNA is five times more likely to remain cleared of Rad51 by Srs2 than the longer T25 ssDNA. The ratio appears to be the same for T20 and T25, reflecting the similar stability of a Rad51 nucleation above T20. If Srs2 is added to the DNA before Rad51, the duration of Srs2 activity before Rad51 formation was substantially longer ( Supplementary Fig. S5a–d ), indicating an enhanced ability of Srs2 to prevent Rad51 binding. Nevertheless, Rad51 filaments eventually reform even under these circumstances and a dynamic exchange between the two states follows as before ( Fig. 5c ). To test whether Srs2 monomer can clear Rad51 filament, we used the protein-tethered assay where DNA prebound with a Rad51 filament was applied to the surface-tethered Srs2 ( Fig. 5e ). We observed a brief low FRET binding followed by high FRET and FRET fluctuations, indicating the binding of a Rad51–ssDNA filament to Srs2, followed by a quick clearance of Rad51- and Srs2-mediated motions on ssDNA, respectively ( Fig. 5f ). This assay offers two unique advantages. First, it enables a direct observation of an Srs2 monomer to clear Rad51. Second, it allows for precise measurement of the time required for an Srs2 monomer to clear a Rad51 filament, δ t ( Fig. 5f ). In agreement with the stability of Rad51 filaments shown above ( Fig. 5d ), the removal time to clear the longest (T20, T25) was 4- to 5-fold higher than the shortest Rad51 filament (T13). The similar fold difference obtained in Fig. 5d,g indicates that the overall filament stability of Rad51 on T20/25 is approximately fivefold higher than that on T13. Srs2 cannot disassemble a RecA filament To examine the specificity of Srs2 in clearing Rad51, we tested its ability to remove RecA filaments. We formed a stable RecA filament [20] and added Srs2 (200 nM). In this case, <5% of the molecules showed FRET fluctuations induced by Srs2, indicating negligible removal of RecA ( Supplementary Fig. S5e ). On the basis of this result, we confirm that Srs2’s repetitive activity is specific for dismantling Rad51 filaments as the anti-recombinase activity of Srs2 requires a direct physical contact with Rad51 [6] , [12] (refs 6,12). In addition, the full-length Srs2 shows the same repetitive movement ( Supplementary Fig. S5f ) and the same pattern of Rad51-clearing activity ( Supplementary Fig. S5g ), indicating that the full-length Srs2 exhibits the same activity as the C-terminal truncation mutant. Srs2 unwinding of DNA is suppressed by Rad51 As a helicase, Srs2 can unwind dsDNA with a flanking 3′-ssDNA tail longer than 12 nucleotides [11] . We asked whether this unwinding activity is modulated by the presence of a Rad51 filament. We confirmed Rad51 formation on dsDNA, as shown before ( Supplementary Fig. S2a–c ). Complete unwinding is expected to result in the loss of the Cy3 (green)-labelled strand because only the other strand (red) is immobilized to the surface ( Fig. 6a,b ). Therefore, the unwinding kinetics was measured by the disappearance rate of the Cy3 (green) signal over time on all DNA constructs ( Fig. 6c ). We counted molecules every 5–10 s after the addition of Srs2 on different regions of the microscope slide, rather than continuous monitoring of one area to minimize photobleaching. Consistent with the previous finding [11] , the rate of unwinding is dependent on the length of the 3′-tail ( Fig. 6d ). In the presence of Rad51, however, the unwinding rate was reduced to the same degree, independent of the tail length ( Fig. 6e,f , Table 1 ), suggesting that Rad51 formed on the duplex DNA is responsible for the inhibitory effect. 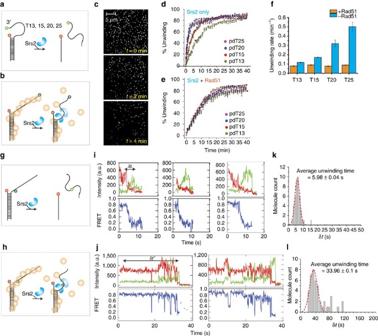Figure 6: Rad51 suppresses Srs2-induced unwinding. (a,b) FRET–DNA constructs with varying tail lengths (T13–T25) without and with Rad51. (c) Fluorescence spots left on surface can be counted for unwinding rate analysis. (d–f) Unwinding rate of Srs2 is substantially lower in the presence of Rad51. Error bars denote s.e.m. based on over 1,000 molecules obtained from three measurements. (g,h) Schematic of unwinding DNA constructs. Cy3 and Cy5 are located near duplex junction such that unwinding will result in FRET decrease. (i,j) Unwinding in the presence of Rad51 is delayed as indicated by slower FRET decrease. (k,l) Histograms and a Gaussian distribution fit show that the Srs2-unwinding duration is about 5–6 times longer in the presence of Rad51. Errors in fit results are in s.e.m. Figure 6: Rad51 suppresses Srs2-induced unwinding. ( a , b ) FRET–DNA constructs with varying tail lengths (T13–T25) without and with Rad51. ( c ) Fluorescence spots left on surface can be counted for unwinding rate analysis. ( d – f ) Unwinding rate of Srs2 is substantially lower in the presence of Rad51. Error bars denote s.e.m. based on over 1,000 molecules obtained from three measurements. ( g , h ) Schematic of unwinding DNA constructs. Cy3 and Cy5 are located near duplex junction such that unwinding will result in FRET decrease. ( i , j ) Unwinding in the presence of Rad51 is delayed as indicated by slower FRET decrease. ( k , l ) Histograms and a Gaussian distribution fit show that the Srs2-unwinding duration is about 5–6 times longer in the presence of Rad51. Errors in fit results are in s.e.m. Full size image Table 1 Unwinding rate with and without Rad51 (min −1 ). Full size table To examine this effect more directly, we prepared a DNA substrate that has two dyes located near the duplex junction ( Fig. 6g,h ). In the absence of Rad51, Srs2 (>20 nM) induces a rapid FRET decrease, as seen in a representative trace ( Fig. 6i ), with the unwinding dwell time (δ t ) of 6 s ( Fig. 6k ). In the presence of a Rad51 filament, however, unwinding is inhibited, as seen by the long delay in the FRET decrease ( Fig. 6j ), yielding an average unwinding time of 34 s ( Fig. 6l ). Next, we employed the Srs2 monomer-tethered assay to test whether monomer can unwind ( Supplementary Fig. S6a ). Over 95% of the binding events showed a stable high FRET ( Supplementary Fig. S6b ), indicating no DNA-unwinding activity. Therefore, we conclude that Srs2 monomers cannot unwind DNA efficiently and that the unwinding seen with immobilized DNA is probably because of higher oligomeric forms of Srs2 or multimers of Srs2 binding to one DNA, consistent with ensemble studies. We have used smFRET to detect the formation of Rad51 filaments on ssDNA with lengths in the 10–20 nucleotide range where the distance change induced by Rad51 binding is detectable by FRET [27] . We observed that Rad51 formed a stable filament on ssDNA as short as 18 nucleotides ( Fig. 1b ). On the basis of the detection of three, four and five steps for Rad51 binding to pdT10, 13 and 15, respectively, we deduced a site size of three nucleotides per Rad51 monomer. Combining the site size with the minimum ssDNA length required for forming a stable Rad51 filament (pdT18), we infer a nucleation size of six Rad51 monomers. These numbers are similar to those inferred for RecA [20] and consistent with the structural resemblance between the two proteins [19] , [21] . It is interesting to note that the FRET transition from 0.8 to 0.65, which represents monomer dissociation near ds/ssDNA junction is substantially less prominent than others in all three TDPs presented ( Fig. 1d ). This pattern possibly arises from the higher stability of a monomer that binds at the ds/ssDNA junction compared with other positions. Therefore, the near-duplex junction positioning of Srs2 represents an ideal target location for an anti-recombinase. Previous studies with hRad51 reported that nucleoprotein filaments grow in multiples of trimers as a stable nucleation cluster [28] . However, this assay was performed on purely dsDNA (λ DNA) on which a Rad51 filament may have a different stability. Similar to our finding, a recent study by Bell et al. [29] demonstrated that RecA filament formation on ssDNA involves primarily monomer and dimer units and the net growth favors the 5′–3′ direction. Although Rad51 binding is expected to be similar to RecA [30] , Rad51-binding directionality has never been demonstrated on a resected DNA mimic with high resolution. In humans, Rad51 binding to resected DNA is controlled by BRCA2 (ref. 31) [31] . In agreement with our finding, the overall net growth directionality for RecA, hRad51 and yeast Rad51 was shown to be 5′–3′ on both ssDNA and dsDNA, although bi-directionality was also demonstrated [20] , [28] , [29] , [32] . To directly monitor the directional bias of yeast Rad51 filament formation, we utilized a recently developed single-molecule assay, smPIFE [14] , [16] . The 5′–3′ assembly was demonstrated in two ways: the difference in the rate of overall signal increase and the shape of the intensity increase ( Fig. 2b,d ). In addition, the larger PIFE effect seen for the 3′-Cy3 is in agreement with our previous finding in which RecA binding to a similar substrate resulted in 3- to 4-fold increase in the fluorescence signal [14] . Previous single-molecule studies have identified numerous helicases that translocate or unwind [16] , [33] , [34] , [35] , [36] , [37] . Two bacterial homologues of Srs2, Rep [34] and PcrA [36] display repetitive translocation that resembles that of Srs2 in two aspects. First, they all exhibit repetitive activity on ssDNA; second, they all involve looping of ssDNA, although the mechanistic details differ. One clear difference is that Srs2 only acts on a small segment of ssDNA near-duplex junction. We propose a model whereby Srs2 stations itself near the junction of ssDNA and dsDNA and repetitively reels in a short segment of ssDNA ( Supplementary Fig. S4m ). We hypothesize that this repetitive activity involves ATP-stimulated conformational changes within Srs2, which results in a periodic tugging of a finite length of ssDNA. We also note that we cannot discern whether this motion involves looping of ssDNA, scrunching or encircling of ssDNA around Srs2. Srs2 is a functionally unique helicase in yeast in that its recruitment is highly specific for the removal of Rad51 filaments [6] , [7] , [38] . As a control, we showed that Srs2 is unable to remove a RecA filament from ssDNA ( Supplementary Fig. S5e ). It is interesting to note that the removal of Rad51 filament formed on shorter fragment of ssDNA requires substantially less time, probably because of instability of the Rad51 filament ( Fig. 5g ). The repetitive motion by Srs2 we demonstrate here is not the dismantling of a Rad51 filament, but what is likely to occur after disruption of the filament. Hence, our findings expand on the previously known role of Srs2’s anti-recombinase function [6] , [7] , [8] , [9] . This repetitive mechanism at the site of a duplex junction can offer two advantages. First, the repetitive nature of activity can effectively maintain ssDNA clear of Rad51 binding. Second, the activity at the duplex junction enables efficient sequestering of ~18–20 nucleotides of ssDNA, which coincides with an ~18-nucleotide-length required for the formation of a stable Rad51 nucleation cluster. Taken together, the Srs2 mechanism we present here ( Fig. 7 ) represents a highly specific activity of an anti-recombinase both in terms of motion and position. We note that the anti-recombinase activity of Srs2 does not prevent Rad51 formation permanently, but only acts to transiently counterbalance Rad51 filament formation. 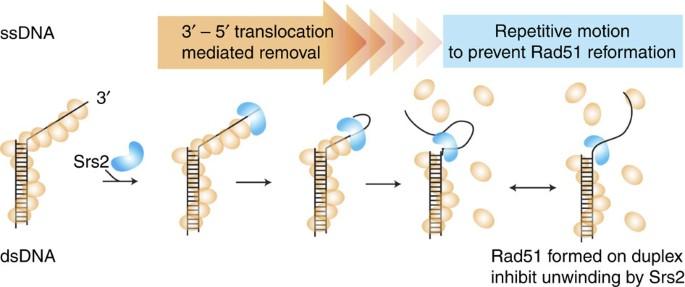Figure 7: Schematic summary of Srs2 motion as an anti-recombinase mechanism for Rad51 clearance. Srs2 first translocates in the 3′–5′ direction along ssDNA to displace Rad51, and then remains bound near the duplex junction and displays repetitive motion on a short segment of ssDNA to prevent Rad51 re-formation. Figure 7: Schematic summary of Srs2 motion as an anti-recombinase mechanism for Rad51 clearance. Srs2 first translocates in the 3′–5′ direction along ssDNA to displace Rad51, and then remains bound near the duplex junction and displays repetitive motion on a short segment of ssDNA to prevent Rad51 re-formation. Full size image The helicase activity of Srs2 is not correlated with its anti-recombinase function [7] , [39] , [40] , whereas the ATP-fuelled translocase activity is required but is not sufficient for Rad51 filament removal [6] , [11] . Furthermore, it has been shown for other SF1 helicases that their translocation and unwinding activities are functionally separable in that enzyme oligomerization is often required for DNA-unwinding activity [41] . We find that monomeric Srs2 can dislodge Rad51 filaments on ssDNA, but cannot unwind dsDNA. Hence, Srs2 monomers are capable of removing Rad51 filaments from ssDNA without unwinding the duplex DNA. This behaviour is thus similar to what has been observed and proposed for Escherichia coli UvrD in its role as an anti-recombinase to remove RecA filaments [37] . Previous studies revealed that Rad51 has a dual role; it targets Srs2 to HR intermediates and triggers ATP hydrolysis within the Rad51 filament, inducing Rad51 dissociation from the DNA [6] . Here we demonstrate yet another role of Rad51 in preventing DNA unwinding by Srs2. In contrast, one study reported that Rad51 enhances Srs2 unwinding [42] . However, this study was performed under very different conditions including the presence of RPA, use of up to a 25-fold higher Srs2 concentration (500 nM) and a DNA with a much longer ssDNA tail (209 nucleotides), all of which may favour the DNA-unwinding reaction. Because of these differences, a direct comparison cannot be made. Our more direct real-time assay shows that in the absence of RPA, Rad51 inhibits the ability of Srs2 to unwind DNA. In conclusion, we present a comprehensive step-by-step process of the roles of Rad51 and Srs2 in the early stages of HR. Our results reveal an exquisite mechanism that controls the balance between the recombinase, Rad51 and the anti-recombinase, Srs2. Oligonucleotides Unlabelled, Cy3-labelled and Cy5-labelled oligonucleotides were purchased from Integrated DNA Technologies (Coralville, IA, USA). Internally labelled oligos contain amino modifier dT subsequently labelled using Cy3 monofunctional NHS esters (GE Healthcare, Princeton, NJ, USA). Briefly, 10 nmol of amino modified oligonucleotides in 20 μl of 50 mM sodium tetraborate buffer (pH 8.5) and 100 nmol of Cy3 NHS ester dissolved in dimethylsulphoxide was added and incubated with rotation overnight at room temperature. The labelled oligonucleotides were purified by ethanol precipitation [43] . DNA sequences pdT(10–70): 5′-GCCTCGCTGCCGTCGCCA-3′+5′-TGGCGACGGCAGCGAGGC-(dT) 10 or (dT) 13 or (dT) 15 or (dT) 18 or (dT) 20 or (dT) 25 or (dT) 30 or (dT) 40 or (dT) 70 -3′; internal amino modifier is represented as (C6 dT), which can be used to label DNA with an internal Cy3 or Cy5 dye. pdT3+17: 5′-GCCTCGCTGCCGTCGCCA-3′+5′-TGGCGACGGCAGCGAGGC-(dT) 3 -(C6 dT)-(dT) 17 -3′; pdT15+(15–35): 5′-GCCTCGCTGCCGTCGCCA-3′+5′-TGGCGACGGCAGCGAGGC-(dT) 15 -(C6 dT)-(dT) 15 or (dT) 25 or (dT) 35 -3′. DNA substrate preparation Partial duplex DNA substrates for immobilized DNA experiments were prepared by mixing the appropriate biotinylated and non-biotinylated oligonucleotides in a 1:2 molar ratio at 10 μM in T50 buffer (50 mM NaCl, 10 mM Tris-HCl (pH 8.0)). Oligonucleotide mixtures were incubated at 95 °C for 2 min followed by slow cooling to room temperature to complete the annealing reaction. Partial duplex DNA substrates for tethered-protein experiments were prepared using non-biotinylated strands of oligonucleotides with the same sequences as those of biotinylated oligos. Proteins The wild-type Rad51 protein and Srs2 truncation mutant Srs2 1–898 (Srs2 CΔ276 ) with a His9 tag at its N terminus were expressed in E. coli Rosetta strains (Novagen) and purified to near homogeneity [6] . The bacterial wild-type RecA protein was purchased from New England Biolabs (Ipswich, MA, USA). Reaction conditions for Rad51 RecA and Srs2 Standard Rad51 reaction buffer was 50 mM Tris-HCl (pH 7.5), 50 mM NaCl, 10 mM MgCl 2 ; standard RecA reaction buffer was 100 mM NaAc, 25 mM Tris-HCl (pH 7.5), 10 mM MgAc, with an oxygen-scavenging system containing 0.8% v/v dextrose, 1 mg ml −1 glucose oxidase, 0.03 mg ml −1 catalase [43] and 2-mercaptoethanol (1% v/v); all items were purchased from Sigma-Aldrich (St Louis, MO, USA). The measurements were performed at room temperature (21±1 °C). ATP (1 mM) was used in all experiments unless otherwise specified. Single-molecule fluorescence assay smFRET and smPIFE measurements were done using a wide-field total internal reflection fluorescence microscope [43] . Cy3 (donor) on DNA was excited using an Nd:YAG laser (532 nM, 75 mW; Coherent CUBE) via total internal reflection. The fluorescence signals from Cy3 and Cy5 were collected through an objective (Olympus Uplan S-Apo; X100 numerical aperture; 1.4 oil immersion) and detected at 100 ms time resolution using an electron multiplying charge-coupled device camera (iXon DU-897ECS0-#BV; Andor Technology). The camera was controlled using home-made C++ program. Single-molecule traces were extracted from the recorded video file using IDL software. Srs2 translocation on ssDNA S. cerevisiae Srs2 was mixed at 5 nM with Rad51 reaction buffer and ATP, and added to a flow chamber that had 100 pM DNA specifically immobilized on a polyethylene glycol (PEG)-coated quartz surface through biotin–neutravidin linkage [44] . ATP concentration varies from 0 to 1 mM for data fitted to Michaelis–Menten equation ( Fig. 3c ). Srs2-unwinding DNA Srs2 (200 nM) was mixed in the Rad51 reaction buffer and applied to surface-immobilized FRET–DNA. Approximately 400–600 single molecules are viewed in one field of image. The disappearance of Cy3 fluorescence was counted as unwound DNA molecules (loss of Cy3 signals) by taking about 20 short movies (5–10 s) taken for over 40 min. Rad51 filament formation Yeast Rad51 was mixed at 1 μM in Rad51 reaction buffer and applied to immobilized DNA. Initially, all DNA molecules displayed high FRET because of ssDNA flexibility. Upon Rad51 formation, high FRET decreased to low FRET. The FRET histograms obtained from thousands of molecules were compiled to represent the population dynamics over time, whereas smFRET traces were analysed further to determine the site size of Rad51 monomers. Removal of Rad51 filament by Srs2 Initially, 1 μM of Rad51 was added to FRET–DNA to complete filament formation. Then, Srs2 and Rad51 were mixed at 200 nM and 1 μM, respectively, in Rad51 reaction buffer and applied to the flow chamber to remove preformed Rad51 filament. Again, the results were analysed at the level of histogram and single-molecule traces. RecA filament formation Bacterial RecA was mixed at 1 μM with RecA reaction buffer and ATP, and added to a flow chamber that had 100 pM specifically immobilized DNA. Tethered Srs2 protein The truncated Srs2 protein, Srs2 CΔ276 has 9 × histadine tags, which are tethered to the PEG-coated quartz surface through neutravidin–biotin–tris–NTA linkage. Biotin–tris–NTA was a generous gift from Professor Paul J. Hergenrother, Department of Chemistry at the University of Illinois Urbana Champaign [45] . For Srs2 translocation experiments, biotin–tris–NTA (20 nM) was mixed with NiCl 2 (50 nM) in T50 buffer (50 mM Tris (pH 7.5), 50 mM NaCl) and incubated on ice for 15 min. The mixture was then added to a flow chamber that already had neutravidin immobilized to the PEG-coated surface, and then allowed to incubate for 10 min at room temperature. Srs2 (0.5–1 nM) in T50 buffer were then added to the flow chamber and incubated for 5 min at room temperature. Finally, non-biotinylated partial duplex DNA substrate in Rad51 reaction buffer and ATP was added to the flow chamber to initiate the reaction. For Srs2 monomer removal of Rad51 filaments, 10 nM of Srs2 was tethered to the quartz surface via neutravidin–biotin–tris–NTA linkage. Non-biotinylated partial duplex DNA substrates were first incubated with 1 μM of Rad51 in Rad51 reaction buffer, and with ATP for 15 min at room temperature before being added to the flow chamber to complete the reaction. Srs2 protein labelling NTA–Atto 647 dye was kindly provided by Professor Robert Tampé, Institute of Biochemistry at Goethe-University Frankfurt [46] . Srs2 and dye were mixed at a ratio of 1:1.5 (5 nM and 7.5 nM, respectively) with Rad51 reaction buffer, ATP, 2 mM dithiothreitol, incubated at room temperature for 5 min, and added to a flow chamber that had 100 pM Cy3-only DNA substrate immobilized. Data analysis Single-molecule traces were analysed using codes written in Matlab. FRET efficiency values were calculated as a ratio between acceptor intensity and total donor and acceptor intensity. For various dwell time analyses peak-to-peak dwell time analysis to obtain δ t was measured manually from individual FRET traces ( Fig. 4d ) within Matlab, and the resulting histograms and fittings were generated using Origin (OriginLab Corporation, Northampton, MA, USA). Binning sizes vary based on the type and range of data collected. Rad51 removal dwell time ( Fig. 6g ) was measured as the time that it took from the appearance of low FRET signal to change to high FRET ( Fig. 6f ). Srs2 loading duration ( Supplementary Fig. S6b,d ) was measured as the time that DNA is occupied by Srs2 before being covered by Rad51 ( Supplementary Fig. S6a,c ). DNA-unwinding time by Srs2 ( Fig. 7k,l ) is measured as the time it took to move from high FRET fluctuations (Srs2-occupying DNA) to low FRET fluctuations before signal disappearance due to DNA unwinding ( Fig. 7i,j ). Overall, ratio measures the time that the DNA spent coated with Rad51 versus free of Rad51. It is calculated by averaging the sum of the individual ratio of each pair of δ t -R (DNA covered with Rad51 filament) and δ t -S (DNA cleared of Rad51 filament) from individual single-molecule traces. δ t is measured as shown in Fig. 6c . Michaelis–Menten kinetics ATP-dependence data for FRET fluctuation dwell times were fitted to the Michaelis–Menten kinetics equation (1) using Origin (OriginLab Corporation). In equation (1), v is the dwell time rate calculated at ATP concentration [ S ]; V max is the maximum dwell time rate achieved at saturating ATP concentration; K m is the amount of ATP required for the reaction to reach half the maximum dwell time rate. How to cite this article: Qiu, Y. et al. Srs2 prevents Rad51 filament formation by repetitive motion on DNA. Nat. Commun. 4:2281 doi: 10.1038/ncomms3281 (2013).